Biomedical photoacoustics beyond thermal expansion using triggered nanodroplet vaporization for contrast-enhanced imaging Since being discovered by Alexander Bell, photoacoustics may again be seeing major resurgence in biomedical imaging. Photoacoustics is a non-ionizing, functional imaging modality capable of high contrast images of optical absorption at depths significantly greater than traditional optical imaging techniques. Optical contrast agents have been used to extend photoacoustics to molecular imaging. Here we introduce an exogenous contrast agent that utilizes vaporization for photoacoustic signal generation, providing significantly higher signal amplitude than that from the traditionally used mechanism, thermal expansion. Our agent consists of liquid perfluorocarbon nanodroplets with encapsulated plasmonic nanoparticles, entitled photoacoustic nanodroplets. Upon pulsed laser irradiation, liquid perfluorocarbon undergoes a liquid-to-gas phase transition generating giant photoacoustic transients from these dwarf nanoparticles. Once triggered, the gaseous phase provides ultrasound contrast enhancement. We demonstrate in phantom and animal studies that photoacoustic nanodroplets act as dual-contrast agents for both photoacoustic and ultrasound imaging through optically triggered vaporization. The generation of sound from the interaction of light with a material is aptly named photoacoustics, a well described physical phenomenon [1] . The combination of photoacoustic and ultrasound imaging provides high spatial resolution images at traditionally ultrasonic depths, a potential benefit for medical imaging [2] , [3] , [4] , [5] . Photoacoustic signal can be generated through four mechanisms including thermal (also referred as thermoelastic) expansion [6] , [7] , vaporization [6] , [7] , photochemical processes [7] , [8] and optical breakdown [6] , [7] . However, in biomedical applications of photoacoustic imaging and sensing, the only biologically safe mechanism to date is thermal expansion. Unfortunately, thermal expansion is one of the least efficient mechanisms of light–sound energy conversion and produces acoustic waves of relatively low amplitude [7] . In thermal expansion-based photoacoustic imaging, sufficiently short laser pulses are absorbed by tissue chromophores, causing localized volume heating, leading to rapid expansion and generation of acoustic pressure waves. With the exception of melanin, haemoglobin and other porphyrins, tissue components have relatively low optical absorption properties, limiting the overall endogenous contrast in photoacoustic imaging. Exogenous contrast in photoacoustic imaging can be achieved through use of contrast agents, such as plasmonic metal nanoparticles [9] , [10] , [11] , [12] . These nanoparticles have optical absorption cross-sections that are orders of magnitude higher than those of tissue components and are generally used to enhance the optical absorption of nanoparticle-labelled tissues. Surface-functionalized nanoparticles also provide molecular functionality with the addition of specific targeting moieties [10] , [11] , [13] . However, the production of photoacoustic transients using these exogenous agents is still governed by thermal expansion, and therefore, the same fundamental limits of this mode of photoacoustic signal generation apply. Exogenous contrast agents have also been designed and developed for ultrasound contrast enhancement. Gas microbubbles, for instance, have long been used in diagnostic ultrasound imaging as highly sensitive, cost effective and biocompatible contrast agents. Owing to their highly scattering acoustic properties and nonlinear interactions with incident ultrasound, microbubbles are used in many clinical applications, including assessment of coronary artery disease, hyperlipidaemia, angiogenesis, inflammation and tumour formation. Microbubbles can also be used to assess therapeutic strategies and to facilitate delivery and release of therapeutic agents based on physical interactions of microbubbles with ultrasound [14] , [15] , [16] . Furthermore, current research is focused on adapting the microbubbles, through surface modifications, cargo encapsulation or attachment, and other modifications, to allow for additional therapeutic applications [17] , [18] , [19] , [20] , [21] , [22] , [23] , [24] . Therefore, microbubbles are a sensitive contrast agent that has diagnostic and therapeutic effects for vascular applications. Microbubbles do have limitations, however. Gas diffusion and biological clearance significantly limit their circulation time and therefore, any potential therapeutic effects through cellular targeting, and chemical or physical treatment. Furthermore, owing to their size (>1 μm), microbubble effects are limited to within the vascular system. The invention of phase shift perfluorocarbon (PFC) liquid droplets and acoustic droplet vaporization (ADV) provided a method to solve both these problems [25] , [26] . Liquid droplets of PFCs, often stabilized with albumin, lipids or polymers, provide a long circulating, triggerable contrast agent. The use of PFCs with boiling points below body temperature (37°C) allow these agents to become superheated and easily vaporize in the presence of pulsed ultrasound with frequencies and pressures in the sub-therapeutic range [27] . However, for tumour imaging, molecular diagnosis and therapy, these particles would have to extravasate out of the vasculature into the tumour interstitial space where cellular interactions could take place. To facilitate these cellular interactions, the phase change agents would have to be smaller than the known endothelial gap junction sizes of up to 800 nm in tumour vasculature. The gap junction size depends strongly on tumour type and location, but sizes between 300 nm to 800 nm have been suggested, and thus, passive accumulation of nanoparticles in tumours, entitled the enhanced permeability and retention effect [28] , can occur with nanoparticles smaller than the junction size [29] , [30] , [31] . While nanoscale PFC droplets can be easily synthesized, their inherent acoustic contrast is minimal (contrast enhancement through Rayleigh scattering of sound) [32] . Large acoustic contrast from these nanoscale PFC droplets occurs only when they undergo a phase transition into a gaseous state. Studies have revealed that ADV requires increased acoustic input as the diameter of the droplets decreases (owing to decreased surface tension [27] and increased boiling point [33] ) and the frequency of the transducer decreases [26] . The extra acoustic input energy is required for ADV as smaller droplets have significantly higher surface tension to overcome. Combined with surface-stabilizing agents (protein, lipids and polymers) these particles become difficult to vaporize with typical diagnostic ultrasound frequencies and pressures. Therefore, acoustic nanodroplet vaporization may require acoustic frequencies and pressures that will also cause unwanted bioeffects [27] . Hence, a methodology to activate PFC nanodroplets without unwanted bioeffects is desired. Here, we have developed an optically activated, nanoscale dual-contrast agent for combined photoacoustic and ultrasound contrast-enhanced imaging. Photoacoustic nanodroplets (PAnDs) consist of a droplet of liquid PFC with a bovine serum albumin (BSA) shell in which optically absorbing nanoparticles have been suspended. These droplets use optical absorption for several purposes including a mechanism to trigger the liquid-to-gas transition of a nanoscale PFC droplet, the production of strong photoacoustic signal through vaporization and prolonged thermal expansion signal via the encapsulated optically absorbing nanoparticles. The resulting gaseous phase of the PFC increases acoustic impedance mismatch for increased ultrasound signal. Therefore, PAnDs comprise three contrast mechanisms simultaneously, offer an environment easily modified for molecular targeting and therapeutic cargo delivery, and provide the opportunity to use the photoacoustic contrast mechanism, vaporization, safely in biological tissues. We discuss synthesis, characterization and utility of PAnDs for photoacoustic and ultrasound imaging. Using hydrogel phantoms, both ultrasound and photoacoustic imaging of the PAnDs was performed to determine and quantify the contrast enhancement from PAnDs. It was demonstrated that PAnDs provide three mechanisms of contrast: vaporization and thermal expansion for photoacoustics, and increased acoustic impedance mismatch for ultrasound. Furthermore, PAnDs were employed in an in vivo murine model to validate the contrast-enhancing effects in highly optically scattering and absorbing tissues. Therefore, vaporization as a photoacoustic phenomenon was introduced at biologically safe levels of laser energy, and the ability of PAnDs to act as an optically triggered dual photoacoustic and ultrasound contrast agent was established. Contrast mechanisms of PAnDs PAnDs are a nano-sized agent consisting of a BSA shell and liquid PFC core, namely perfluoropentane with a boiling point of 27°C, in which specially capped plasmonic noble metal nanoparticles have been encapsulated ( Fig. 1a ). PAnDs are stable because while their nanoscale size increases surface tension, the BSA shell dramatically lowers the surface tension and prevents coalescence, thus preventing premature vaporization of superheated PFC from both clinically relevant imaging ultrasound fields and elevated temperatures (up to 50°C for 200 nm diameter droplets). Therefore, pulsed laser irradiation is used to activate this contrast agent, that is, to remotely trigger the phase transition of PFC. The PAnDs are vaporized when encapsulated plasmonic nanoparticles, such as gold nanorods, absorb electromagnetic energy from the laser, providing localized heating well over the required vaporization temperature of PFC [34] (steps 1–2 in Fig. 1b ). In addition, a high-frequency pressure wave is generated at the surface of the plasmonic nanoparticles. Together, heat and pressure provide the conditions required to nucleate a liquid-to-gas phase transition of PFC, and the PAnD undergoes a vaporization, which overcomes the surface tension of the BSA coating (step 3 in Fig. 1b ). The photoacoustic transient produced via vaporization is substantially larger than subsequent transients produced from the expelled plasmonic nanoparticles, which undergo thermal expansion under continued pulsed laser irradiation (steps 4–5 in Fig. 1b ). Furthermore, the resulting gaseous phase also provides increased acoustic impedance mismatch between gas bubbles and the surrounding medium (step 6 in Fig. 1b ), providing, in essence, optically triggered ultrasonic contrast enhancement. Overall, PAnDs provide several types of contrast for two imaging modalities: vaporization and thermal expansion for photoacoustic imaging, and gas-tissue acoustic impedance mismatch for ultrasound imaging. 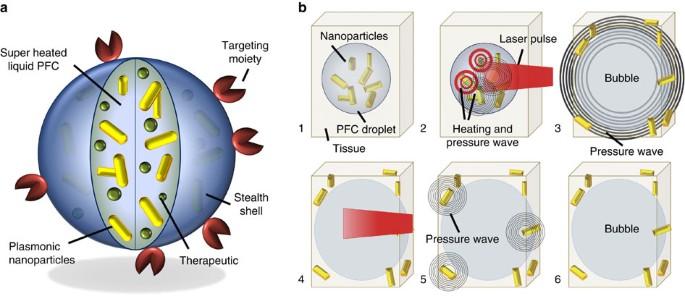Figure 1: PAnDs concept and mechanisms. (a) Diagram depicting the dual-contrast agent concept—photoacoustic droplet consisting of plasmonic nanoparticles suspended in encapsulated PFC (a superheated liquid at body temperature) and capped with a BSA shell. PAnDs may further contain therapeutic cargo and be surface functionalized for molecular targeting and cell–particle interactions. (b) Step-by-step diagram of remote activation of PAnDs, providing photoacoustic signal via two mechanisms: vaporization of PAnDs (steps 2–3) and thermal expansion caused by plasmonic nanoparticles (steps 4–5). The resulting gas microbubble of PFC (step 6) provides US contrast due to acoustic impedance mismatch between gas and the surround environment. Figure 1: PAnDs concept and mechanisms. ( a ) Diagram depicting the dual-contrast agent concept—photoacoustic droplet consisting of plasmonic nanoparticles suspended in encapsulated PFC (a superheated liquid at body temperature) and capped with a BSA shell. PAnDs may further contain therapeutic cargo and be surface functionalized for molecular targeting and cell–particle interactions. ( b ) Step-by-step diagram of remote activation of PAnDs, providing photoacoustic signal via two mechanisms: vaporization of PAnDs (steps 2–3) and thermal expansion caused by plasmonic nanoparticles (steps 4–5). The resulting gas microbubble of PFC (step 6) provides US contrast due to acoustic impedance mismatch between gas and the surround environment. Full size image Characterization of PAnDs After synthesis of PAnDs via an oil-in-water emulsion technique (see Methods ), several approaches were used to characterize PAnDs. First, cryogenic transmission electron microscopy (cTEM) illustrates the spherical PFC droplets containing plasmonic gold nanorods [35] with an overall size, controlled to ~200 nm using an extruding technique ( Fig. 2a ). cTEM imaging also confirms that the overall diameter and extent of nanoparticle loading can be controlled during the synthesis process. 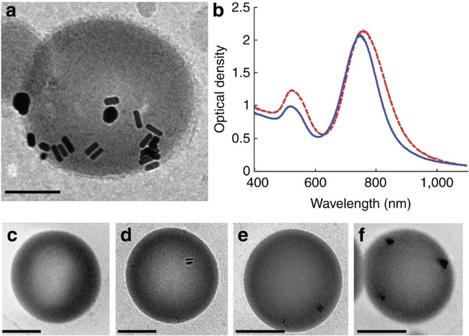Figure 2: PAnDs. (a) cTEM image of PanDs-containing nanorods—plasmonic nanoparticles with high optical absorption cross-section. Scale bar, 100 nm. (b) Extinction spectra of as-prepared nanorods and nanorods with a modified surface required for incorporation into The red line represents the optical density spectrum of the gold nanorods as synthesized, while the blue line represents the spectrum of the nanorods after organic surface modification. (c–f) cTEM images of unloaded PAnD and PAnDs with varying compositions (including (dande) loading with gold nanorods and (f) silver nanoplates with various sizes (200 nm in panelcandd, and 400 nm in panelseandf). Scale bars incandd, 100 nm. Scale bars ineandf, 200 nm. Figure 2c displays a 200-nm PAnD purposefully without any nanoparticle loading, while Figure 2d displays a 200-nm droplet designed to have a lesser extent of gold nanorod loading. Figure 2e displays a PAnD sized to 400 nm with gold nanorod loading. Furthermore, different types of nanoparticles, including iron-oxide particles, gold nanospheres or silver nanoplates ( Fig. 2f ), and dyes can be incorporated into PAnDs. Second, spectrophotometry was used to ensure that the surface modification process did not alter the specifically tuned optical properties of the gold nanorods. The 'as prepared' and 'modified' gold nanorod spectra indicated only very small differences, and therefore the optical properties were not significantly altered during the ligand exchange process [36] . Finally, dynamic light scattering was used to confirm sizing diameters. It was found that the size distributions closely corresponded with the size of the extruder membranes used. For a particular imaging or therapeutic application, PAnDs can be customized allowing for adjustments of size, loading and surface functionalization. Figure 2: PAnDs. ( a ) cTEM image of PanDs-containing nanorods—plasmonic nanoparticles with high optical absorption cross-section. Scale bar, 100 nm. ( b ) Extinction spectra of as-prepared nanorods and nanorods with a modified surface required for incorporation into The red line represents the optical density spectrum of the gold nanorods as synthesized, while the blue line represents the spectrum of the nanorods after organic surface modification. ( c–f ) cTEM images of unloaded PAnD and PAnDs with varying compositions (including ( d and e ) loading with gold nanorods and ( f ) silver nanoplates with various sizes (200 nm in panel c and d , and 400 nm in panels e and f ). Scale bars in c and d , 100 nm. Scale bars in e and f , 200 nm. Full size image Photoacoustic and ultrasound imaging in vitro Combined photoacoustic and ultrasound imaging demonstrates the contrast enhancement provided by PAnDs. Experiments were performed using a block-shaped hydrogel made out of an optically transparent, 10% polyacrylamide gel, homogenously laden with 200-nm PAnDs containing gold nanorods (see Methods for details). The hydrogel-based phantom was placed in a water tank and imaged before, during and after laser irradiation using a 7-MHz ultrasound transducer array positioned at the top of the phantom. An optical beam generated from a tunable pulsed laser system (780-nm wavelength, 5–7-ns pulse duration, 10 -Hz pulse repetition rate, 5.0 mJ cm −2 ) was focused sequentially onto the phantom at varying depths from 1–2 cm. Photoacoustic transients were collected at 3.3 Hz for 30 s. The initial photoacoustic signal corresponding to the vaporization of PAnDs was substantially higher than the subsequent transients corresponding to thermal expansion. When comparing the photoacoustic images ( Fig. 3a ), the vaporization signal had higher intensity than the thermal expansion. Furthermore, photoacoustic intensity measured over time (that is, as the pulsed laser irradiation continues) presented a rapid decay of the signal magnitude ( Fig. 3b ) corresponding to the expected difference in the mechanisms of photoacoustic signal generation. The initial signal collected before laser irradiation illustrates the level of noise inherent in the imaging system. Once the laser was turned on, there was a dramatic increase in photoacoustic signal magnitude due primarily to the rapid, laser-triggered vaporization of PAnDs. As laser irradiation continued, and the supply of PAnDs was depleted, the photoacoustic signal decayed to its steady-state level corresponding to the thermal expansion of the expelled gold nanorods. In biological tissue, unlike the case of the hydrogel phantom, thermal expansion from endogenous optical absorbers will also contribute to the photoacoustic signal. 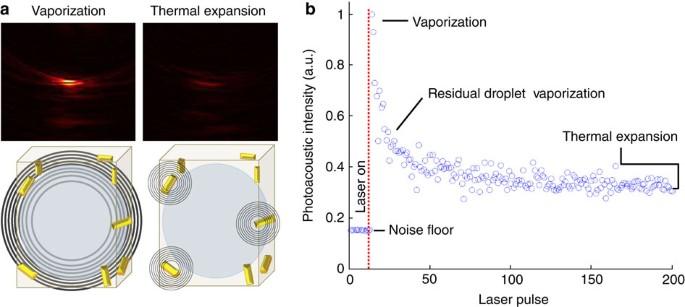Figure 3: Photoacoustic contrast enhancementin vitro. (a) Photoacoustic images reconstructed using vaporization-based and thermal expansion-based signals captured at one location. Each spot size is 1 mm. The schematic diagrams below indicate the associated mechanisms of photoacoustic signal generation. Qualitatively, the vaporization-based image has stronger photoacoustic signal and higher SNR compared with the traditional, thermal expansion-based photoacoustic image. (b) Magnitude of pressure transients, measured as the pulsed laser irradiation continues (that is, over time), indicating the difference in photoacoustic signal produced by vaporization and thermal expansion mechanisms. The lowest level of signal before laser irradiation is indicative of system noise. Once the pulsed laser irradiation is on, the magnitude of photoacoustic signal is initially dominated by PAnD vaporization. The later, steady-state level of photoacoustic signal is attributed to thermal expansion caused by gold nanorods. In this experimental setup, 50% of the droplets are disrupted by the eighth laser pulse. This value, however, is variable depending on several factors, including droplet size, extent of nanoparticle loading, laser fluence, and optical properties of the surrounding environment. Figure 3: Photoacoustic contrast enhancement in vitro . ( a ) Photoacoustic images reconstructed using vaporization-based and thermal expansion-based signals captured at one location. Each spot size is 1 mm. The schematic diagrams below indicate the associated mechanisms of photoacoustic signal generation. Qualitatively, the vaporization-based image has stronger photoacoustic signal and higher SNR compared with the traditional, thermal expansion-based photoacoustic image. ( b ) Magnitude of pressure transients, measured as the pulsed laser irradiation continues (that is, over time), indicating the difference in photoacoustic signal produced by vaporization and thermal expansion mechanisms. The lowest level of signal before laser irradiation is indicative of system noise. Once the pulsed laser irradiation is on, the magnitude of photoacoustic signal is initially dominated by PAnD vaporization. The later, steady-state level of photoacoustic signal is attributed to thermal expansion caused by gold nanorods. In this experimental setup, 50% of the droplets are disrupted by the eighth laser pulse. This value, however, is variable depending on several factors, including droplet size, extent of nanoparticle loading, laser fluence, and optical properties of the surrounding environment. Full size image Using the same phantom and experimental setup, several more locations (28 total) underwent pulsed laser irradiation in sequence where photoacoustic signals were captured for each laser pulse. These locations were strategically placed to 'write' the letters 'U' and 'T.' The reconstructed photoacoustic images of the phantom ( Fig. 4a ) confirm that under the same laser fluence, vaporization of PAnDs results in a stronger photoacoustic signal compared with nanorod-assisted photoacoustic signal generated by thermal expansion alone. The vaporization-based photoacoustic image displays a signal-to-noise ratio (SNR) of 7.3 dB, while the thermal expansion-based photoacoustic image displays a SNR of 1.3 dB. Furthermore, the average photoacoustic signal increase from all 28 positions is ~13 times, or 22 dB, higher than the thermal expansion signal, with a maximum reaching 66 times, or 37 dB, higher. Therefore, laser-induced vaporization of the PAnDs produced a significantly stronger photoacoustic signal than that of thermal expansion. We measured the photoacoustic signal generated by the vaporization of the PFC in PAnDs (first laser pulse, steps 2–3 in Fig. 1b ) and the thermal expansion of the nanorods that were expelled into the surrounding environment (subsequent laser pulses, repeated steps 5–6 in Fig. 1b ). The change in photoacoustic signal magnitude was significant ( Fig. 3b )—vaporization of PAnDs resulted in a strong photoacoustic signal that was measurably higher compared with photoacoustic transients produced by thermal expansion. Importantly, the results of the phantom experiment also indicated that the same amplitude of the photoacoustic signal can be obtained with lower concentrations of gold nanorods inside of PAnDs compared with nanorods alone ( Fig. 4b ). Overall, vaporization of the PAnD contrast agent provided stronger photoacoustic signal as compared with the thermal expansion photoacoustic phenomena mediated by plasmonic nanoparticles. 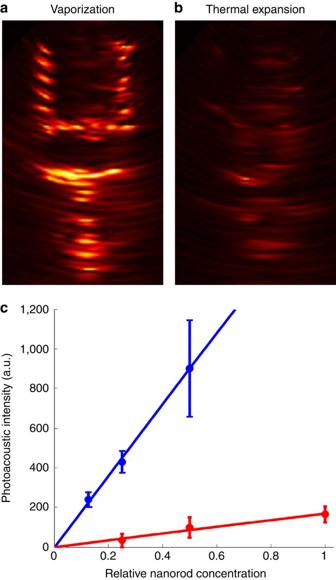Figure 4: Photoacoustic imagingin vitro. (a) Photoacoustic images of the laser beam drawn letters 'U' and 'T' reconstructed using vaporization-based signals. Both letters stand 1.2 cm tall and 0.5 cm wide. (b) Photoacoustic image of the thermal expansion-based signals over the same area asa. The vaporization-based image has stronger signal and higher SNR compared with the traditional, thermal expansion-based photoacoustic image. (c) Analysis of photoacoustic signal amplitude from PAnDs (blue line) and gold nanorods alone (red line) reveals that for the same concentration of gold nanorods, photoacoustic signal amplitude from 200-nm PAnDs is an order of magnitude higher than the nanorod-assisted photoacoustic signal.n= 3. Error bars indicate 1 s.d. Figure 4: Photoacoustic imaging in vitro . ( a ) Photoacoustic images of the laser beam drawn letters 'U' and 'T' reconstructed using vaporization-based signals. Both letters stand 1.2 cm tall and 0.5 cm wide. ( b ) Photoacoustic image of the thermal expansion-based signals over the same area as a . The vaporization-based image has stronger signal and higher SNR compared with the traditional, thermal expansion-based photoacoustic image. ( c ) Analysis of photoacoustic signal amplitude from PAnDs (blue line) and gold nanorods alone (red line) reveals that for the same concentration of gold nanorods, photoacoustic signal amplitude from 200-nm PAnDs is an order of magnitude higher than the nanorod-assisted photoacoustic signal. n = 3. Error bars indicate 1 s.d. Full size image Furthermore, once the vaporization of PAnDs was initiated, the generated gaseous phase of the PFC had a significant acoustic impedance mismatch with the surrounding environment, thus acting as an ultrasound contrast agent ( Fig. 5 ). 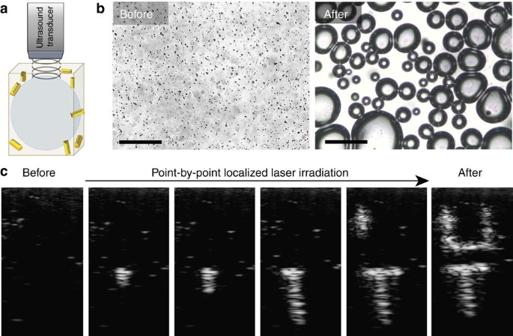Figure 5: Ultrasound contrast enhancementin vitro. (a) Depiction of the gas phase of a PAnD after laser-triggered vaporization has occurred. These microbubbles provide significant acoustic impedance mismatch between the PFC gas and the surrounding environment. (b) Optical images of a hydrogel with PAnDs before laser exposure and after laser exposure. Individual droplets are expected to create bubbles approximately five times the diameter of the original droplet. The larger bubbles are due to rapid coalescence of smaller bubbles. Scale bars represent 50 μm. (c) Sequential ultrasound frames captured as the laser irradiation produced desired pattern in the phantom. The image before laser irradiation illustrates that the ultrasound field alone does not activate PAnDs (that is, does not initiate the liquid-to-gas transfer of the PFC). As PAnDs are irradiated with laser beam at corresponding positions, the microbubbles are locally triggered, resulting in ultrasound contrast enhancement. Each individual spot is ~1 mm, with the final letters standing 1.2 cm tall and 0.5 cm wide. Images are in 20-dB scale. Figure 5a shows how the resulting gaseous PFC will act to increase ultrasonic contrast by increased acoustic impedance mismatch in the phantom. The liquid-to-gas transition of PAnDs is illustrated in the optical images in Figure 5b . The left panel of Figure 5b contains light microscopy images of PAnDs suspended in a hydrogel block. The hydrogel was irradiated with a pulsed laser beam and additional optical images were taken (right panel in Fig. 5b ). The large size of gas bubbles appearing in Figure 5b were due to coalescence of several individual microbubbles in close proximity. During the photoacoustic imaging experiment ( Fig. 4a ), ultrasound signals were collected before and after each laser application. With point-by-point optical laser activation of PAnDs, the ultrasound contrast appears at the corresponding positions of the laser–PAnD interaction ( Fig. 5c ) due to an ultrasound pulse backscattered from PanD-generated microbubbles. Therefore, vaporization of the PFC in PAnDs also provides increased ultrasound contrast. Figure 5: Ultrasound contrast enhancement in vitro . ( a ) Depiction of the gas phase of a PAnD after laser-triggered vaporization has occurred. These microbubbles provide significant acoustic impedance mismatch between the PFC gas and the surrounding environment. ( b ) Optical images of a hydrogel with PAnDs before laser exposure and after laser exposure. Individual droplets are expected to create bubbles approximately five times the diameter of the original droplet. The larger bubbles are due to rapid coalescence of smaller bubbles. Scale bars represent 50 μm. ( c ) Sequential ultrasound frames captured as the laser irradiation produced desired pattern in the phantom. The image before laser irradiation illustrates that the ultrasound field alone does not activate PAnDs (that is, does not initiate the liquid-to-gas transfer of the PFC). As PAnDs are irradiated with laser beam at corresponding positions, the microbubbles are locally triggered, resulting in ultrasound contrast enhancement. Each individual spot is ~1 mm, with the final letters standing 1.2 cm tall and 0.5 cm wide. Images are in 20-dB scale. Full size image Photoacoustic and ultrasound imaging in vivo While PAnDs produced high levels of contrast enhancement in in vitro phantoms studies, it is important to test their performance in an in vivo setting. A murine model was adapted for in vivo studies. Under ultrasound guidance, an anesthetized nu/nu mouse was injected with 50 μl of PAnDs at a concentration of 10 8 PAnDs ml −1 into the pancreas, which resides under the spleen at ~5–7 mm of depth from the skin surface. The spleen represents a highly optically absorbing organ owing to its high blood content. Imaging through the blood-laden spleen and at depth in the pancreas represents a challenge for PA imaging applications, and therefore it was chosen as an imaging target to exhibit the contrast-enhancing capabilities of PAnDs. Using a Vevo2100 (VisualSonics, Inc.) ultrasound imaging system equipped with a 40 MHz, 256 element transducer, ultrasound pulse-echo signals and photoacoustic transients were collected. Photoacoustic transients were generated under pulsed laser irradiation (10 Hz, 5–7-ns pulse duration, 14 mJ cm −2 ) using a tunable laser system operating at 780 nm (the peak optical absorption of the gold nanorods encapsulated within PAnDs). For more details, please see Methods section. Photoacoustic images were collected for 475 laser pulses (that is, 475 photoacoustic frames). Initially, the laser beam was blocked from irradiating the animal to prevent unrecorded vaporization of PAnDs and to determine the noise level of the imaging system. Upon radiation, the photoacoustic signal within the region of interest corresponding to injected PAnDs was initially very strong and, as the pulsed laser irradiation continued, it decayed to the level corresponding to superposition of signals from the expelled nanorods and endogenous thermal expansion ( Fig. 6a ). The vaporization signal was 4.3 dB higher than that given by the nanorod and endogenous chromophores combined. Based on control experiments (described in Methods), using the equivalent number of nanorods as encapsulated in the injected PAnDs, the increase of signal generated by the nanorods alone was ~1.9 dB, for a total of 6.0 dB increase in signal generation using PAnDs. 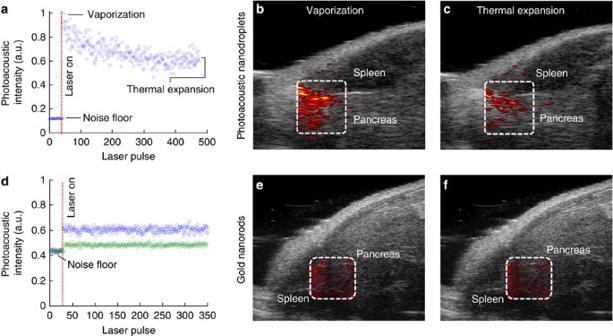Figure 6: Ultrasound contrast enhancementin vivo. (a) Graph depicting the average photoacoustic intensity within the region of interest corresponding to the injected PAnDs, indicated by boxes in panelband panelc. Upon pulsed laser irradiation, photoacoustic signal is high and then, with continued pulsed laser irradiation, decays to a steady-state level of thermal expansion-based photoacoustic signal related to the expelled nanorods and endogenous chromophores. Vaporization signal over thermal expansion signal represents a 4.3-dB increase. (b) Combined ultrasound and photoacoustic image of the peak photoacoustic signal generated from the rapid phase transition of the PAnDs. (c) Combined ultrasound and photoacoustic image representing photoacoustic signal generated from expelled gold nanorods and endogenous chromophores. Each frame is 20.4 mm wide by 12.8 mm tall. ultrasound is in 20-dB scale. In this experimental setup, ~50% of the droplets are disrupted by the 60th laser pulse. (d) Graph displaying changes of photoacoustic signals during continued pulsed laser irradiation before and after an injection of only gold nanorods. The green circles represent photoacoustic signal of the endogenous photoabsorbers in the mouse tissues. Blue circles represent the photoacoustic signal owing to thermal expansion caused by both the endogenous photoabsorbers and the injected gold nanorods. It is important to note that there was no significant change of these signals as laser irradiation continued, unlike those signals created by PAnDs. The injection of gold nanorods constituted a 1.9-dB increase in signal. (e,f) Combined photoacoustic and ultrasound images of mouse cross-section and injection site of gold nanorods immediately after the laser was turned on (first laser pulse) and at the end of the laser pulsing (last laser pulse). Note that there is insignificant difference between these images (e,f), suggesting a static signal production via thermal expansion. Each image is 12.2 mm wide by 10.8 mm tall. ultrasound image is displayed using 20-dB scale. The corresponding combined photoacoustic and ultrasound images in Figure 6b,c illustrate the peak photoacoustic signals corresponding to vaporization of PAnDs and thermal expansion. As evident from Figure 6 , the photoacoustic signal produced by the initial vaporization is much stronger than the signal produced by thermal expansion. Figure 6: Ultrasound contrast enhancement in vivo . ( a ) Graph depicting the average photoacoustic intensity within the region of interest corresponding to the injected PAnDs, indicated by boxes in panel b and panel c . Upon pulsed laser irradiation, photoacoustic signal is high and then, with continued pulsed laser irradiation, decays to a steady-state level of thermal expansion-based photoacoustic signal related to the expelled nanorods and endogenous chromophores. Vaporization signal over thermal expansion signal represents a 4.3-dB increase. ( b ) Combined ultrasound and photoacoustic image of the peak photoacoustic signal generated from the rapid phase transition of the PAnDs. ( c ) Combined ultrasound and photoacoustic image representing photoacoustic signal generated from expelled gold nanorods and endogenous chromophores. Each frame is 20.4 mm wide by 12.8 mm tall. ultrasound is in 20-dB scale. In this experimental setup, ~50% of the droplets are disrupted by the 60th laser pulse. ( d ) Graph displaying changes of photoacoustic signals during continued pulsed laser irradiation before and after an injection of only gold nanorods. The green circles represent photoacoustic signal of the endogenous photoabsorbers in the mouse tissues. Blue circles represent the photoacoustic signal owing to thermal expansion caused by both the endogenous photoabsorbers and the injected gold nanorods. It is important to note that there was no significant change of these signals as laser irradiation continued, unlike those signals created by PAnDs. The injection of gold nanorods constituted a 1.9-dB increase in signal. ( e , f ) Combined photoacoustic and ultrasound images of mouse cross-section and injection site of gold nanorods immediately after the laser was turned on (first laser pulse) and at the end of the laser pulsing (last laser pulse). Note that there is insignificant difference between these images ( e , f ), suggesting a static signal production via thermal expansion. Each image is 12.2 mm wide by 10.8 mm tall. ultrasound image is displayed using 20-dB scale. Full size image PAnDs versus gold nanorod efficiency An in vivo experiment was undertaken to determine how effective PAnDs are in producing photoacoustic contrast as compared with the traditional contrast agent, plasmonic gold nanorods alone. To define the exact amount of nanorods encapsulated in the injected amount of PAnDs in the in vivo experiment, several samples were analysed using spectrophotometry. The spectrum of highly scattering and absorbing PAnDs loaded with gold nanorods was compared with the optically scattering spectra of empty PAnDs to estimate the absorption of nanorods encapsulated in PAnDs. A solution of nanorods with polyethylene glycol grafted to their surface was diluted in water until the optical density matched that of the encapsulated nanorods. Using an anesthetized Nu/Nu mouse and the same imaging setup used in the in vivo experiment, baseline photoacoustic and ultrasound images were taken to evaluate the endogenous contrast inherent in a mouse spleen and pancreas. The noise floor of photoacoustic imaging system was evaluated using these images. Then, 50 μl of the diluted nanorod solution, for a total of ~5×10 8 nanorods, was injected using the same protocol as the in vivo experiment. The animal was imaged and changes in photoacoustic intensity during continued laser irradiation were analysed, as displayed in Figure 6d–f . A comparison of photoacoustic signal from thermal expansion caused by endogenous photoabsorbers and the photoacoustic signal from thermal expansion caused by both the endogenous photoabsorbers and the injected gold nanorods revealed that the associated signal increase is 24%, or 1.9 dB. The percentage difference in signal provided by an absolute number of nanorods can be used to determine the overall photoacoustic signal enhancement caused by PAnDs above the endogenous contrast of the animal with the same absolute number of nanorods encapsulated. Furthermore, it is pertinent to note that under the laser fluence used in our experiments, the gold nanorods remained thermodynamically stable [37] and, therefore, do not exhibit photoacoustic signal change with laser irradiation. Furthermore, nanorods alone do not induce vaporization comparable to PAnDs. The photoacoustic and ultrasound signals as the laser irradiated the sample at the first/last photoacoustic frames collected are depicted in Figure 6e–f . As expected, there was no change in these images with continuing laser irradiation. PAnDs not only produce significant enhancement of photoacoustic contrast in a mouse model but PAnDs also provide significant ultrasound contrast once injected and remotely triggered. 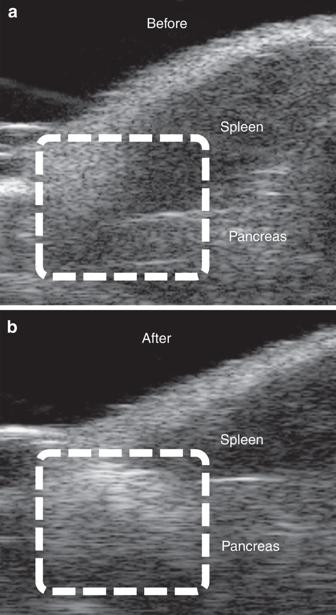Figure 7: Ultrasound contrast enhancementin vivo. (a) US image of a mouse cross-section before injection of PAnDs displaying the location of the spleen and pancreas. (b) US image of the same cross-section after the direct injection and laser activation of PAnDs. The boxes in both images identify the region of interest where PAnDs were injected. The activated PAnDs resulted in an ~29-dB increase over the native contrast. Both panels are 13.5 mm wide by 18.1 mm tall, and are in 20-dB scale. Ultrasound images of a mouse cross-section before injection of PAnDs and after the laser activation injected PAnDs are shown in Figure 7 . Owing to the dynamic respiratory/cardiac motion and the nature of internal organs, ultrasound contrast varies owing to migration of PAnDs and bubbles in and out of the imaging plane, coalescence of bubbles, gas diffusion and delayed vaporization of PAnDs. The peak increase of ultrasound contrast was 3.1 dB over post-injection images, and ~29 dB over native ultrasound images. This experiment demonstrates optically triggered, ultrasound contrast enhancement in a living, biological system. Figure 7: Ultrasound contrast enhancement in vivo . ( a ) US image of a mouse cross-section before injection of PAnDs displaying the location of the spleen and pancreas. ( b ) US image of the same cross-section after the direct injection and laser activation of PAnDs. The boxes in both images identify the region of interest where PAnDs were injected. The activated PAnDs resulted in an ~29-dB increase over the native contrast. Both panels are 13.5 mm wide by 18.1 mm tall, and are in 20-dB scale. Full size image The developed contrast agent, namely PAnDs, can be remotely triggered to provide both ultrasound and photoacoustic contrast enhancement through vaporization and gas bubble formation. As such, the PAnDs are naturally applicable for combined photoacoustic and ultrasound imaging. Overall, PAnDs provide three mechanisms of contrast enhancement: a one-time, laser-induced vaporization of the PFC within PAnDs to produce photoacoustic contrast; long-term thermal expansion induced by the plasmonic nanoparticles absorbing laser energy and yielding photoacoustic contrast; and acoustic impedance mismatch between the surrounding tissues and the microbubbles-containing PFC in gaseous phase producing ultrasound contrast. These three contrast mechanisms have been demonstrated to produce high levels of contrast enhancement both in phantom and live animal experiments, confirming the feasibility of the PAnDs as an optically triggered, dual-contrast agent for clinical photoacoustic and ultrasound imaging. These contrast mechanisms were not only demonstrated in a hydrogel phantom, but also in a biological environment to show efficacy in tissues. Compared with phantoms, tissue experiments are associated with several challenges, including increased optical absorption and scattering, a high level of background photoacoustic signal due to endogenous chromophores, such as melanin and haemoglobin, and higher laser fluence required to image at sufficient depth. The in vivo studies were critical to demonstrate the applicability of PAnDs to overcome challenges provided by imaging in a biological setting. Furthermore, these studies suggest that the use of PAnDs for photoacoustic imaging in clinical applications is feasible. Beyond inducing large photoacoustic transients, the gaseous phase of the PFC serves a secondary function as a remotely triggered ultrasound contrast agent. Indeed, the PAnDs have high surface tension that prevents them from vaporizing under clinically relevant ultrasound fields and slight variations of temperatures. Conversely, micro-sized PFC droplets do not experience the same surface tension, burst easily, but have a limited ability to enter interstitial space owing to their larger size compared with PAnDs [26] , [38] . Therefore, until exposure to laser irradiation and optical absorption of the laser energy by the plasmonic nanoparticles occurs, the PAnDs remain inert and virtually undetectable by conventional ultrasound imaging. The ultrasound images in Figure 5c are shown in a non-scattering background, and therefore the ultrasound signals are easy to visualize. In a scattering media such as tissue, as depicted by the in vivo mouse study, the contrast is not as dramatic. However, various acoustic techniques such as nonlinear [39] or second harmonic [40] acoustic spectroscopy may be implemented to further enhance the contrast. Therefore, the PAnD-based platform provides a nano-scale, biocompatible (see Methods for details) and efficient contrast agent for both photoacoustic and ultrasound imaging. In addition, the developed platform can utilize broad spectrum of electromagnetic wave 'triggers' by incorporating the corresponding thermally responsive particles within the PFC droplets. PAnDs have several benefits for biological imaging owing to their unique physical properties. As vaporization provides stronger photoacoustic signal than thermal expansion, by employing PAnDs, a smaller number of noble metal nanoparticles can be used in biological and clinical applications of photoacoustic imaging, reducing the potential toxic effects of plasmonic particles [41] . Furthermore, in biological tissues increased fluence is required to image at sufficient depth. At fluences as low as 8 mJ cm −2 , gold nanorods can become thermodynamically unstable and this can significantly change their optical properties [37] . PAnDs produce higher photoacoustic signal with only limited laser exposure, as indicated in our phantom and mouse imaging, effectively rendering the thermal stability of nanorods of limited concern. This increased signal can even aid in providing photoacoustic imaging at depths beyond what is obtainable using traditional plasmonic contrast agents and dyes. Finally, regardless of the initial surface fluence of the light delivery, within several centimeters of depth in tissue, the fluence has greatly decreased. As exhibited by phantom experiments, PAnDs require only minimal energy (a fluence of a few mJ cm −2 ) to activate into their contrast-enhancing state, making them able to provide contrast deep within tissues. Recent studies [42] have revealed that photoacoustic imaging at alternative wavelengths, specifically 1064 nm, minimizes endogenous contrast of the tissues, enabling increased imaging depth. Furthermore, the ANSI laser exposure standard also dramatically increases to ~100 mJ cm −2 in this infrared region [43] . PAnDs can be easily tuned to vaporize at a desired wavelength by changing the aspect ratio of the nanorod, or encapsulating a different plasmonic particle that has peak absorption at the desired wavelength. Therefore, PAnDs are specifically designed to be used in biological contrast-enhancing applications. Beyond its use as a dual-contrast agent, PAnDs are adaptable for a variety of applications ranging from fundamental biomedical studies to medical diagnostic and therapeutic applications. First, they can be loaded with organic chemotherapeutics that would be selectively released at the location of laser activation [44] , [45] , [46] . In order to use chemotherapeutics properly, an initial injection of contrast agent without the drug may be used to image (that is, locate and diagnose) the pathology, and then a second, drug-loaded injection could be used to safely introduce a therapeutic agent. Furthermore, the surface of the PAnD can be modified to allow for molecular targeting of specific biological targets [47] , [48] ( Fig. 1a ). Finally, a plethora of other therapeutic effects could be optimized using PAnDs, including targeted image-guided photothermal therapy [49] , drug delivery and release [24] , vessel occlusion [26] , [38] and cell membrane sonoporation effects from vaporization [50] . Synthesis of PAnDs Synthesis of the remotely triggered PAnDs occurred in three steps. First, plasmonic nanoparticles were synthesized and surface modified to allow solubility in organic solvents. Second, the surface-modified plasmonic nanoparticles were resuspended in liquid PFC. Finally, the liquid PFC was emulsified with a BSA solution, and the PAnDs were sized using a lipid mini extruder. This procedure created stable, nano-sized PAnDs to be used for ultrasound and photoacoustic imaging. Methods for synthesis of different plasmonic nanoparticles were adopted from the corresponding original synthesis procedures [35] , [36] , [51] . Silver nanoplates were synthesized through reduction of silver ions by ascorbic acid [12] . The nanoparticle of focus, gold nanorods, was synthesized first using a slightly modified seed-mediated growth method [35] . To make the gold nanorods and silver nanoplates soluble in an organic environment, a two-step ligand exchange method [51] was adopted with slight modifications. Specifically, 5 ml of thiolated poly (ethylene glycol) (mPEG-SH, 5000 Da, Laysan Bio) in water (2.0 mg ml −1 ) and 5 ml of as synthesized gold nanorods (40 nm by 10 nm) were sonicated for 2 min and left to react at room temperature for 2 h. The solution was centrifuged at 10,000 rcf for 10 min and the supernatant was removed. The nanorods were redispersed in 5 ml of tetrahydrofuran (THF, Sigma Aldrich). Next, 5 ml of ethanolic dodecanethiol (Sigma Aldrich, 1.0 mg ml −1 ) was added to the THF-nanorod solution and sonicated at room temperature for 30 min. The temperature was increased to 50°C for an additional 60 min of sonication. The solution was then left to rest overnight. The solution was then centrifuged at 10,000 rcf for 10 min and the supernatant was discarded. The dodecanethiol-capped nanorods were resuspended in chloroform. To synthesize the photoacoustic droplets, first 1 ml of as prepared gold nanorods in chloroform were placed into a 7-ml glass scintillation vial. The organic solvent was completely evaporated, leaving dried nanorods on the bottom of a glass vial. Then, 0.25 ml of liquid perfluoropentane (PFP, Fluoromed, Inc.) was added to the vial and sonicated for 2 min using a bath sonicator. Next, 2 ml of BSA (Sigma) in saline was added (0.2 mg ml −1 ), and the two solutions were sonicated to produce a coloured (pink), opaque emulsion of the PAnDs in the water phase. The PAnDs were then extruded using a lipid extrusion system through polycarbonate membranes (Avanti Polar Lipids) with a 200-nm pore size. This extrusion yielded a 10 8 PAnD per ml solution. Three methods were used to characterize the PAnDs. First, ultraviolet to visible spectrophotometry (DU640, Beckman Coulter) was used to study the optical extinction of the PAnDs and incorporated plasmonic nanoparticles ( Fig. 2b ). PAnDs were synthesized as described above, diluted and optical density was measured in a 1-cm plastic cuvette. Second, dynamic light scattering (DelsaNano C, Beckman Coulter) was used to determine the size distribution of the nanocarrier agent. PAnDs at synthesized concentration were measured and the resulting size distribution correlated with the pore size of the extruder filter used to size the PAnDs, 200 nm for these experiments. Finally, cTEM (FEI Tecnai G2 F20, FEI) was used to image the PAnDs ( Fig. 1b,d ). This method allows visualization of an intact PAnD and the metal nanoparticles within. As prepared PAnDs were diluted by 100 times and placed on holey carbon grids and vitrified in liquid ethane using a Vitrobot (FEI) with a 1.0-s blotting time. Samples were rapidly transferred to liquid nitrogen and stored until imaging. Nanoparticle encapsulation was verified by sample stage rotation to view the sample at 0°, 45° and −45°. These three forms of nanocarrier contrast agent characterization allowed for study of both physical and optical characteristics. Photoacoustic and ultrasound imaging in vitro PAnDs were incorporated into a 10% polyacrylamide (Sigma Aldrich) hydrogel phantom crosslinked with a 0.1% w/v ammonium persulfate (Sigma Aldrich) in a 1:20 volume ratio of agent to polyacrylamide solution for a final concentration of 5.5×10 6 PAnDs ml −1 (optical image in Fig. 5b ). The phantom was positioned in a water bath and imaged from the top using a 7 MHz, 1.4 cm aperture, 128 element, linear array transducer. A tunable laser system (optical parametric oscillator pumped by a Q-switched pulsed Nd:YAG laser, Opotek) operating at 780-nm wavelength light, 5.0 mJ cm −2 pulse energy, 10 Hz pulse repetition rate and 5–7-ns pulse duration was used to irradiate the phantom perpendicular to the imaging plane at 28 different locations for 60 s. Ultrasound radiofrequency signals were collected before and after each laser irradiation application. Photoacoustic radiofrequency signals were collected during laser irradiation. Ultrasound and photoacoustic images were reconstructed retrospectively from the captured data. Specifically, the radiofrequency ultrasound signals collected at each transducer were Hilbert transformed and beamformed, and then the amplitude of the signal was scan converted and displayed using either a linear (photoacoustic) or logarithmic (ultrasound) scale (20 dB). To form photoacoustic images displaying photoacoustic response from all 28 laser beam positions, photoacoustic images at each individual position were normalized and added to produce the final photoacoustic image. Concentration versus photoacoustic signal amplitude study To determine the photoacoustic signal produced from varying concentrations of PAnDs as compared with the equivalent concentration of gold nanorods, experiments were conducted using 40 nm by 10 nm nanorods and PAnDs incorporating the same nanorods. The results of this study are displayed in Fig. 4c . A thin, 0.2 mm diameter, glass tube was suspended in a water cuvette, and known concentrations of either PAnDs (containing of 0.25, 0.125 and 0.0625 fraction of the original, as prepared concentration of nanorods) or nanorods alone (1.0, 0.5 and 0.25 of the original concentration) were injected into the sample tube. A pulsed (10 Hz, 5–7-ns pulse duration) laser beam was used to irradiate the sample with 780-nm light at 5 mJ cm −2 from the side. Photoacoustic signal was collected using a 7.5 MHz, single-element ultrasound transducer positioned above the sample in the water tank. Peak signal was averaged for three samples per condition, and plotted using error bars representing 1 s.d. Cytotoxicity study PAnDs, prepared as previously described (10 8 PAnDs ml −1 ), were used for this study. PAnDs (5 ml) were sterilized under UV light for 20 min. The sterilized PAnDs were then centrifuged and resuspended in sterile cell media at overall concentrations of up to 1.2 mg ml −1 . A 96-well plate was seeded with 10,000 MPanc96 pancreatic cancer cells per well, and incubated at 37°C and 5% CO 2 for 24 h before further incubation with PAnDs. The media (Dulbecco's modified Eagle's medium with 10% fetal bovine serum and 1% pen-strep) was aspirated, and the new media containing varying concentrations of PAnDs was placed in the predetermined wells. The plate was incubated for another 24 h at 37°C and 5% CO 2 . An initial absorbance was measured using a plate reader (Synergy HT, BioTek) at 490 nm. Next, 20 μl of 3-(4,5-dimethylthiazol-2-yl)-5-(3-carboxymethoxyphenyl)-2-(4-sulfophenyl)-2H-tetrazolium (MTS) was added to each well and incubated at 37°C and 5% CO 2 for 2 h. The mitochondrial activity in viable cells reduces the MTS to a formazan product that has a peak optical absorbance at 490 nm. A final absorbance reading was taken. The initial absorbance reading of each well was subtracted from the final reading to determine the relative viability values. A one-way analysis of variance was used to determine statistically significant different mean viabilities between the control wells and the wells incubated with varying concentrations of PAnDs. With a resulting P -value of 0.8756 for the highest concentration of 1.2 mg ml −1 PAnDs, the null hypothesis that the absorbance means are the same cannot be rejected. Therefore, as the absorbance means between control wells and wells with PAnDs were not statistically significantly different, the PAnDs exhibited no cytotoxicity on the cells as determined by this MTS assay. Photoacoustic and ultrasound imaging in vivo PAnDs were synthesized as previously described at a concentration of 10 8 PAnDs ml −1 with approximately ten gold nanorods per droplet as determined by spectrophotometry and cTEM, and then sized to 400 nm using a lipid miniextruder. A female, 3-month-old, nu/nu mouse (Charles River Laboratory) was anesthetized using 1.5% isoflurane and 2.5% oxygen following proper animal care and use protocols. (Animal handling and care complied with the Guide for the Care and Use of Laboratory Animals (1996). Animal study protocol was approved by The University of Texas at Austin Institutional Animal Care and Use Committee (IACUC).) The spleen and pancreas were located using a Vevo2100 ultrasound imaging system (VisualSonics) equipped with a 40 MHz, 256-element array transducer. To generate photoacoustic transients, the tissue was irradiated with a laser beam (780-nm wavelength, 5–7-ns pulses, 10-Hz pulse repetition frequency and 14 mJ cm −2 fluence) generated by a Nd:YAG Q-switched pulsed laser pumping an optical parametric oscillator (Newport—Spectra Physics). Control ultrasound and photoacoustic images were taken before nanoparticle injection. Using a needle, 100 μl of an equal volume mixture of PAnDs and Matrigel (BD Biosciences), used to prevent high levels of migration of the PAnDs away from the injection site, were injected into the pancreas of the mouse under ultrasound image guidance. Matrigel has peak absorption at ~461 nm, and, as confirmed in previous experiments, does not produce appreciable photoacoustic signal in response to 780-nm laser irradiation. After the injection, photoacoustic signals were recorded before and during pulsed laser irradiation (475 laser pulses). The ultrasound and photoacoustic images were reconstructed off-line, and displayed using a linear (photoacoustic) or logarithmic (ultrasound) scale. How to cite this article: Wilson, K. et al . Biomedical photoacoustics beyond thermal expansion using triggered nanodroplet vaporization for contrast-enhanced imaging. Nat. Commun. 3:618 doi: 10.1038/ncomms1627 (2012).